One-step pipetting and assembly of encoded chemical-laden microparticles for high-throughput multiplexed bioassays One quantitative liquid handling method in conventional assay processes is pipetting, which delivers a precise volume of one sample at a time. As this process becomes laborious and time-consuming as the number of samples increases, researchers in individual laboratories need a way to conduct large-scale assays in a reasonable amount of time and at an affordable cost. Here we report a novel handling technique of chemical substances termed ‘partipetting’, which allows the one-step pipetting of various chemical-laden hydrogels. We pipette and assemble various types of encoded chemical-laden microparticles in microwell arrays in parallel. The combination of this heterogeneous particle chip and a cell chip induces the release of the chemicals from the hydrogels and, eventually, the chemicals treat the targets. Based on bioassay applications using partipetting, we show its capability in large-scale bioassays, without the need for high-throughput bioassay resources, owing to a reduction in the assay costs and time. Advances in a wide range of assay technologies have accelerated the discovery process for novel biochemical and pharmaceutical substances [1] , [2] , [3] , [4] . Prescreened candidate compounds and combinations of compounds may have high diagnostic or therapeutic potential for specific applications; thus, identifying these candidates in an efficient manner has assumed great importance in the biomedical industry. Unfortunately, the discovery and verification processes that necessitate the investigation of chemical molecules addressing a broad range of requirements involve considerable reagent costs and reaction times. Thus, these processes tend to be conducted only by large pharmaceutical companies and a few resourceful research institutes. Therefore, individual laboratories, which cannot afford exorbitant assay costs and high-priced equipment, have increased the demand for new strategies to provide more equal access to large-scale bioassays with reasonable costs and time requirements. Quantitative liquid handling is one of the essential operations in the assay process and critically influences assay cost and time. Manual pipetting is predominantly used to deliver a precise volume of a sample to conventional microtiter plates, and researchers in individual laboratories usually deliver the reagents to the assay platform by manually pipetting one liquid sample at a time. This routine process becomes very laborious and time consuming as the number of test samples increases. If the researcher wants to design a quantitative assay investigating many types of chemicals, then the same number of separate pipetting events will be required for each type of chemical. Additionally, for a conventional pipette, the minimum handling volume of the liquid is limited to the microlitre level, which causes a significant, costly waste of targets, compounds and reagents. The pipetting technique has been automated to make this process less labour-intensive. Automated liquid handlers dispense a selected quantity of reagent into a designated container in a rapid manner and have led to significant advances in dispensing throughput over the past few years compared with manual pipetting. However, in addition to the equipment expense and complicated operation, the dramatic increase in throughput directly results in a dramatic increase in reagent costs because automated systems consume the same amount of reagents as does the manual pipetting method. The reagent cost is the main obstacle for many small laboratories that want to expand their assays to a large scale. In terms of reaction volumes, microfluidics-based assays can be used to implement numerous reactions in nanolitre-sized reactors, which is much smaller than in pipetting-based assays [5] , [6] , [7] , [8] , [9] . Unfortunately, implementing a microfluidic device in large-scale multiplexed assays remains challenging, mainly because of the increased complexity of the interface for material delivery, for example, plumbing tubes and pumps. An important question is how to provide an opportunity for researchers in individual laboratories to conduct large-scale bioassays in a reasonable amount of time and, more importantly, at an affordable cost. To that end, a new strategy should facilitate reaction volume reduction and parallel and heterogeneous liquid handling. In this article, we present a multiplexed bioassay method based on a novel handling procedure of chemical substances and name this process ‘partipetting’. This technique represents one-step pipetting together with directed assembly of encoded chemical-laden hydrogels. Here the hydrogel microparticles, which have two-dimensional (2D) graphical barcodes and can hold sub-nanolitre volumes of chemicals, are first prepared for each chemical. Then different encoded hydrogel particles loaded with chemicals are mixed to form a pooled ECM library. This step facilitates the simultaneous handling of many encoded chemical-laden microparticles (ECMs), despite being mixed in the same vial, by virtue of the particles’ individual identifying characteristics. To illustrate the potential of our technique, we performed multiplexed and combinatorial cytotoxicity assays of osteosarcoma cells (U2OS) with various anticancer drugs and confirmed that the partipetting-based assay method is compatible with a conventional assay technique. To perform this type of testing, we simply pipette various ECMs into the assay platform. The ECMs are then subjected to heterogeneous directed assembly in separate microwells. The unique code on the particles facilitates the identification of each ECM, even though numerous ECMs are randomly assembled in the microwells. Face-to-face attachment of this heterogeneous particle chip to a target cell chip induces the release of chemical substances from the encoded hydrogels and a subsequent reaction with the cells. With only a single pipetting event on a single chip, we can conduct ~5,500 simultaneous cytotoxicity assays, which is equivalent to an individual assay with 57 conventional 96-well microtiter plates. The real value of the partipetting technique is in the feasibility of large-scale quantitative bioassays in individual laboratories, without any aid from a high-priced automated liquid handling station. Therefore, we anticipate that our technique will enable individual researchers to perform multiplexed and high-throughput bioassays with greatly reduced processing time, reagent costs and labour. ECMs and partipetting Partipetting, as we define it, is a single pipetting operation for the simultaneous directed assembly of many different ECMs in separate reaction wells in a microfabricated microwell plate, thus implying ‘pipetting of encoded particles’. 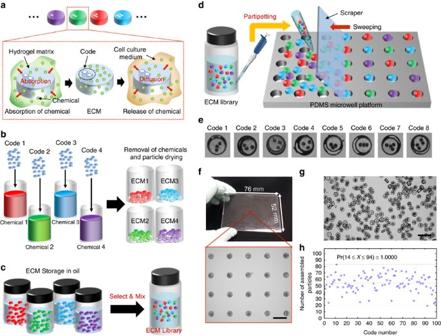Figure 1: The concept of partipetting as a cell-based bioassay platform. (a) Encoded chemical-laden microparticles (ECMs). Each code represents a type of chemical absorbed in the hydrogel matrix. The ECMs selected for the bioassay are mixed together in a single pool, forming an ECM library. The inset (red dashed box) shows absorption of chemicals into the hydrogel matrix and release of chemicals from the ECM. The chemicals absorbed into the hydrogels are released into the buffer by diffusion when the hydrogel comes into contact with either the cell culture medium or buffer solution. (b) ECM preparation. Initially, chemicals are absorbed into the hydrogel matrix through nonspecific absorption. After the absorption of chemicals, excess solution is removed, and the ECMs are dried. (c) ECM library preparation. Dried ECMs are stored in mineral oil, and selected ECMs are mixed together in a single pool for pipetting. (d) The concept of partipetting. Combining the words ‘particles’ and ‘pipetting’ results in the term ‘partipetting’. As the term suggests, encoded microparticles in oil are pipetted into a microwell platform with carrier fluid and assembled in microfabricated wells by sweeping the substrate using a scraper. A single pipetting of various ECMs results in heterogeneity of the assay platform. (e) ECMs with eight different codes in microwells. Each ECM (180 μm in diameter) is positioned in a single well (200 μm in diameter). The code represents the chemical absorbed into the particle. (f) Bright-field microscopy of encoded microparticles assembled in microwells. (g) The number-coded microparticles used inFig. 1f, from codes 00–99. (h) Code distribution of the assembled microparticles. Initially, particles were loaded into a microwell platform, with identical quantities per code, to empirically determine whether partipetting produces an even code distribution after assembly. The number of assembled particles per code is between a minimum of 19 and a maximum 83, with a mean value of 54 (green dotted line, blue dotted line and red line inFig. 2h, respectively). Scale bars, 500 μm. This method reduces not only the number of processes needed for chemical substance loading, owing to the simultaneous handling of numerous microparticles, but also the assay cost, owing to a dramatic reduction in the total volume of handed chemicals ( Supplementary Table 1 ). Figure 1 shows the concept of ‘partipetting’. The partipetting-based bioassay starts with the fabrication of ECMs, which involves the photopolymerization of hydrogel microparticles ( Supplementary Fig. 1 ), followed by loading of chemical substances. In other words, the ECMs are photopolymerized hydrogels with a unique code representing the type of chemical that is physically entrapped within the polymer matrix. The hydrogel microparticles can hold a sub-nanolitre volume of chemicals, which is much less than in other delivery methods of chemicals [10] , [11] , [12] , [13] , and these hydrogels are individually identifiable by their 2D graphical barcodes [14] , [15] , [16] , [17] , [18] , [19] . To prepare the ECM library, each chemical is loaded into a correspondingly encoded hydrogel, and these ECMs are stored in a shrunken and dried form. The ECM library is simply generated by mixing selected ECMs into a single pool, as shown in Fig. 1a–c . This library is maintained in an oil solution, such as a solution containing mineral or silicon oil, until a release cue ( Supplementary Fig. 2 ). When a ECM touches a liquid buffer, such as cell culture medium, chemical substances can immediately diffuse from the hydrogel matrix to the outer buffer solution [20] , [21] ( Fig. 1a inset). Figure 1: The concept of partipetting as a cell-based bioassay platform. ( a ) Encoded chemical-laden microparticles (ECMs). Each code represents a type of chemical absorbed in the hydrogel matrix. The ECMs selected for the bioassay are mixed together in a single pool, forming an ECM library. The inset (red dashed box) shows absorption of chemicals into the hydrogel matrix and release of chemicals from the ECM. The chemicals absorbed into the hydrogels are released into the buffer by diffusion when the hydrogel comes into contact with either the cell culture medium or buffer solution. ( b ) ECM preparation. Initially, chemicals are absorbed into the hydrogel matrix through nonspecific absorption. After the absorption of chemicals, excess solution is removed, and the ECMs are dried. ( c ) ECM library preparation. Dried ECMs are stored in mineral oil, and selected ECMs are mixed together in a single pool for pipetting. ( d ) The concept of partipetting. Combining the words ‘particles’ and ‘pipetting’ results in the term ‘partipetting’. As the term suggests, encoded microparticles in oil are pipetted into a microwell platform with carrier fluid and assembled in microfabricated wells by sweeping the substrate using a scraper. A single pipetting of various ECMs results in heterogeneity of the assay platform. ( e ) ECMs with eight different codes in microwells. Each ECM (180 μm in diameter) is positioned in a single well (200 μm in diameter). The code represents the chemical absorbed into the particle. ( f ) Bright-field microscopy of encoded microparticles assembled in microwells. ( g ) The number-coded microparticles used in Fig. 1f , from codes 00–99. ( h ) Code distribution of the assembled microparticles. Initially, particles were loaded into a microwell platform, with identical quantities per code, to empirically determine whether partipetting produces an even code distribution after assembly. The number of assembled particles per code is between a minimum of 19 and a maximum 83, with a mean value of 54 (green dotted line, blue dotted line and red line in Fig. 2h , respectively). Scale bars, 500 μm. Full size image Generally, researchers in individual laboratories deliver chemicals to a platform by manually pipetting samples one at a time. Thus, they rarely have the opportunity to perform large-scale assays because of limited resources. However, in the partipetting process, the ECMs are pipetted from a pooled ECM library into a microwell plate, and with a single pipetting event, these microparticles are assembled in many separate microwells to form a variable particle chip. We have adopted a scraper-assisted assembly method to deliver the microparticles to the microwells and to remove excess microparticles remaining on the substrate [22] , [23] . The composition of a particle chip depends on the random distribution of encoded microparticles on the substrate. Thus, the code distribution of microparticles should be determined to guarantee the multiplexing capability of this platform. We hypothesized that the assembled microparticles in our particle chip have a code distribution analogous to that of the loaded particles in the microwell plate and verified this concept experimentally by partipetting 100,000 microparticles with 100 different codes in a 76 × 52 mm-sized chip with 7,523 effective microwells ( Fig. 1f ). The microparticles were loaded into a microwell plate, with identical quantities of each code, or ~1,000 particles per code ( Fig. 1g ), and we counted the number of particles assembled in the particle chip to analyse the code distribution via partipetting. As shown in the code distribution displayed in Fig. 1h , we had a minimum of 19 microparticles, a maximum of 83 particles and an average of 54 assembled particles per code in the particle chip. The assembly yield was 72%, which corresponded to a total of 5,416 microwells filled with particles. We estimated the theoretical probability of an assembled particle being in the chip per code to be 1 in 14–94 wells, using a binomial distribution ( Supplementary Methods ). Therefore, the counted number of assembled particles across all codes fits in the estimated range. This result signifies that the assembled ratio of the microparticles with 100 different codes was nearly analogous to the loaded ratio, as we expected. Chip preparation and assay procedure In a cell-based assay using the partipetting approach, we prepare a particle chip with assembled ECMs and a separate cell chip with seeded target cells to prevent premature release of chemical substances. These two chips are combined face-to-face to permit the release of chemicals and subsequent exposure to the cells only when the user wants to perform an assay, as shown in Fig. 2a . After the combined chips have been incubated in an appropriate environment for the assay, the chips are separated, and the assay results are analysed. 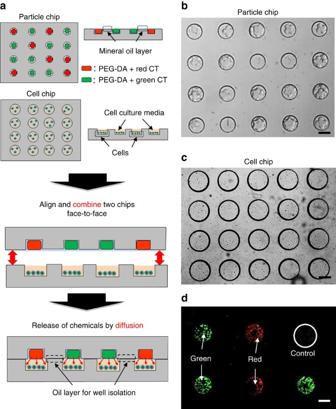Figure 2: Partipetting-based heterogeneous cell staining. (a) Schematic diagram of the chemical substance release process. Particle chip and cell chip for heterogeneous cell staining. Cell-staining dyes (red and green CT) are loaded into the photopolymerized poly(ethylene glycol) diacrylate (PEG-DA) particles. The particle chip and the cell chip are aligned and combined face-to-face to facilitate the release of chemical substances. Target cells in the cell chip react with the chemicals released from the particle chip. The chemicals are released by diffusion through the contact surface between an ECM and cell culture medium. The mineral oil layer from the particle chip prevents the cross-contamination of chemicals (Supplementary Fig. 6). (b) Image of a particle chip. Encoded microparticles are assembled in a particle chip. Each microwell in a particle chip has a diameter of 200 μm and a depth of 60 μm. (c) Image of a cell chip. A cell chip is filled with seeded cells. Each microwell has a diameter of 500 μm and a depth of 300 μm. (d) Fluorescence image of cells heterogeneously stained via partipetting. Scale bars, 300 μm. Figure 2: Partipetting-based heterogeneous cell staining. ( a ) Schematic diagram of the chemical substance release process. Particle chip and cell chip for heterogeneous cell staining. Cell-staining dyes (red and green CT) are loaded into the photopolymerized poly(ethylene glycol) diacrylate (PEG-DA) particles. The particle chip and the cell chip are aligned and combined face-to-face to facilitate the release of chemical substances. Target cells in the cell chip react with the chemicals released from the particle chip. The chemicals are released by diffusion through the contact surface between an ECM and cell culture medium. The mineral oil layer from the particle chip prevents the cross-contamination of chemicals ( Supplementary Fig. 6 ). ( b ) Image of a particle chip. Encoded microparticles are assembled in a particle chip. Each microwell in a particle chip has a diameter of 200 μm and a depth of 60 μm. ( c ) Image of a cell chip. A cell chip is filled with seeded cells. Each microwell has a diameter of 500 μm and a depth of 300 μm. ( d ) Fluorescence image of cells heterogeneously stained via partipetting. Scale bars, 300 μm. Full size image For particle chip preparation, ECMs are partipetted into a 30 × 30 mm microfabricated polydimethylsiloxane (PDMS) microwell platform. Partipetting involves the delivery of various ECMs from a single pool to the well platform, followed by the directed assembly of the particles in the microwells. During the partipetting process, oil is used as a carrier liquid to assemble the particles smoothly and to prevent the cross-contamination of chemicals ( Supplementary Fig. 3 ). When a lubricating solution is not used, the dried hydrogels tend to be easily broken by the scraper during the assembly process. Figure 2d shows cell staining with dye-laden microparticles assembled in a microwell platform. Although all of the various particles are randomly assembled in the microwell plate, each particle can be easily identified by its shape code. Note that a single ECM fits into a single microwell because the size and height of the microparticle are slightly smaller than those of a microwell. Each microparticle has a diameter of 180 μm and a thickness of 60 μm, resulting in a sub-nanolitre volume capacity to contain chemicals, and a microwell has a diameter of 200 μm and a depth of 80 μm. This dimension matching prevents the unwanted stacking of microparticles, thus minimizing the overloading of microparticles in a single well. As a result, because the partipetting-based approach reduces the laborious repetition of heterogeneous chemical substance introduction into the microwell plates by exploiting the ECM library, various types of chemicals can be handled within few pipetting events. The preparation of the cell chip involves dispensing 4 ml of cells in culture medium into the microwell plate (10 5 cells per ml), and the dispersed target cells then settle on the bottom of the wells by gravity. After settling of the cells for 30 min, we sweep over the surface of the plate using a cell scraper to eliminate excess cells from the substrate [23] , [24] . Figure 2c shows the target cells seeded in microwells after overnight incubation, with an average of 167±47 cells per well. Each microwell in the cell chip has a diameter of 500 μm and a depth of 300 μm, which is larger than the particle, providing sufficient culture medium to the cells. The prepared particle chip and cell chip are eventually combined in the release step of chemical substances, forming a sandwich structure [13] , [25] , [26] . During this process, the chemical-laden microparticles come into contact with the cell culture medium, and diffusion-mediated release of chemicals from the hydrogel matrix begins immediately after the two chips are combined ( Supplementary Figs 4 and 5 ). During the release process of chemical substances, it is important to ensure that each well is completely isolated from the other wells to prevent the cross-contamination of chemicals. The oil used in the partipetting process functions as an isolating material, as shown in Fig. 2a . The oil layer on the contact surface between the cell chip and the particle chip prevents the mixing of chemicals between wells, thereby allowing independent and isolated release of chemicals ( Supplementary Fig. 6 ). In the proof-of-concept experiment shown in Fig. 2 , two types of the cell-staining dye CellTracker (CT) were loaded into shape-encoded hydrogels to show heterogeneous cell staining via the partipetting method. The star-shaped microparticle contained a green-staining dye, and the circle-shaped microparticle contained a red-staining dye. Target cells seeded in the microwells were incubated overnight, and, as shown in Fig. 2d , the cells in each microwell were successfully labelled with the corresponding cell-staining dye. Multiplexed cytotoxicity assay We conducted a multiplexed cytotoxicity assay to illustrate the potential of the partipetting-based bioassay. In particular, we performed a cell viability assay to observe the activity of anticancer drugs against U2OS human osteosarcoma cells. The ECM library included eight anticancer drugs: camptothecin (CPT), sodium salicylate (SS), paclitaxel (PTX), auranofin (AF), PKF118-310 (PKF), and three combinatorial drugs containing different concentrations of CPT and SS. Before conducting the cytotoxicity test, an evaluation of the exact concentration of anticancer drugs released from the ECMs is required because the chemicals are loaded into the hydrogels via absorption during the ECM fabrication process and released once in contact with cell culture medium. The molecular concentration of the released anticancer drugs was measured using a UV spectrophotometer ( Supplementary Fig. 7 ). The light absorbance of several known concentrations of each anticancer drug was measured to generate a reference calibration curve, after which the absorbance of the anticancer drugs released from the ECMs into deionized (DI) water was measured to determine the released anticancer drug concentrations. Table 1 shows the loading and released concentrations of eight different anticancer drugs into and from the ECMs, respectively. The drug release rate is defined as the percentage ratio of the released concentration to the loading concentration of an anticancer drug, and this rate depends on the molecular weight of each anticancer drug. For example, PTX (MW=853.91) released 3.3% of its loading concentration, and CPT (MW=348.4) released 13.6% of its loading amount. The final concentrations of the anticancer drugs delivered to the target cells were identical to the released concentrations from the ECMs. Table 1 Loading and released concentrations of anticancer drugs. Full size table After the drug release profiles had been characterized using a UV spectrometer, we prepared the particle chip with eight types of ECMs and the cell chip with U2OS cells, combined these two chips face-to-face and allowed them to react for 24 h in an incubator. Note that the culture medium in the cell chip should be changed to serum-free culture medium before combining the two chips to enhance the drug efficacy against the cells. After the incubation, the particle chip was removed, and the cell chip was treated with an FITC Annexin V Apoptosis Detection Kit to assess cell death by apoptosis or necrosis. FITC-annexin V binds to phosphatidylserine, which is translocated to the outer cell membrane, producing green fluorescence. Based on annexin V binding, we can identify apoptotic cells, that is, the cells that have reacted with the anticancer drugs. In addition, propidium iodide (PI), a membrane-impermeable red fluorescent DNA-staining dye, labels necrotic cells that have damaged membranes. Thus, the assay labels the cells in the following way: viable cells are annexin − /PI − , early apoptotic cells are annexin + /PI − and late apoptotic or necrotic cells are annexin + /PI + . 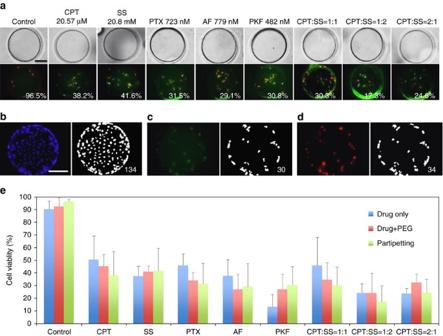Figure 3: A multiplexed cytotoxicity assay using cancer cells and eight anticancer drugs. (a) Multiplexed cytotoxicity assay by partipetting. Eight anticancer drugs (camptothecin (CPT), sodium salicylate (SS), paclitaxel (PTX), auranofin (AF), PKF118-310 (PKF), and three combinations of different concentrations of CPT and SS) released from ECMs were delivered to U2OS cancer cells seeded in a cell chip. The cells were treated with an FITC Annexin V Apoptosis Detection Kit after 24 h. The mean values of the measured cell viability in each condition are denoted in the fluorescence microscopy images. (b–d) Cell counting via image processing to measure viability. (b) Fluorescence image of total cells in a single microwell (DNA staining with Hoechst 33342) and binary image of counted cells. (c) Fluorescence image of apoptotic cells (FITC-annexin V binding to externalized phosphatidylserine) and binary image of counted apoptotic cells. (d) Fluorescence image of necrotic cells (DNA staining by PI) and binary image of counted necrotic cells. (e) Comparison of cell viabilities obtained by a conventional technique and the partipetting technique. The blue bars in the graph represent the viabilities of cells treated with drugs alone in pipetting-based conventional microtiter plates, serving as reference data. The red bars represent the viabilities of cells treated with the same types and concentrations of anticancer drugs but in contact with photopolymerized PEG-DA microparticles in microtiter plates, used to confirm that the PEG-DA microparticles do not alter drug efficacy. The green bars represent cell viabilities obtained using the partipetting-based assay platform, and the data are within a maximum of ±17% of the conventional assay data (n≥10; the values are means±s.d.). Scale bars, 200 μm. Figure 3a shows microwell images of cells treated with drugs delivered via partipetting. The control group in this experiment consisted of cell-containing wells matched with wells containing no ECMs. Figure 3: A multiplexed cytotoxicity assay using cancer cells and eight anticancer drugs. ( a ) Multiplexed cytotoxicity assay by partipetting. Eight anticancer drugs (camptothecin (CPT), sodium salicylate (SS), paclitaxel (PTX), auranofin (AF), PKF118-310 (PKF), and three combinations of different concentrations of CPT and SS) released from ECMs were delivered to U2OS cancer cells seeded in a cell chip. The cells were treated with an FITC Annexin V Apoptosis Detection Kit after 24 h. The mean values of the measured cell viability in each condition are denoted in the fluorescence microscopy images. ( b – d ) Cell counting via image processing to measure viability. ( b ) Fluorescence image of total cells in a single microwell (DNA staining with Hoechst 33342) and binary image of counted cells. ( c ) Fluorescence image of apoptotic cells (FITC-annexin V binding to externalized phosphatidylserine) and binary image of counted apoptotic cells. ( d ) Fluorescence image of necrotic cells (DNA staining by PI) and binary image of counted necrotic cells. ( e ) Comparison of cell viabilities obtained by a conventional technique and the partipetting technique. The blue bars in the graph represent the viabilities of cells treated with drugs alone in pipetting-based conventional microtiter plates, serving as reference data. The red bars represent the viabilities of cells treated with the same types and concentrations of anticancer drugs but in contact with photopolymerized PEG-DA microparticles in microtiter plates, used to confirm that the PEG-DA microparticles do not alter drug efficacy. The green bars represent cell viabilities obtained using the partipetting-based assay platform, and the data are within a maximum of ±17% of the conventional assay data ( n ≥10; the values are means±s.d.). Scale bars, 200 μm. Full size image We quantified cell viability using the fluorescent images of anticancer drug-treated U2OS cancer cells. To count the total number of cells, including both viable and dead cells, we used a cell membrane-permeable DNA-staining dye (Hoechst 33342, Invitrogen). Figure 3b shows DNA-stained U2OS cells in microwells, including both viable and dead cells, after 24 h of drug treatment. We determined the total number of cells to be 134 using image processing. Of a total of 134 cells, there were 30 green-fluorescent cells in the stage of apoptosis ( Fig. 3c ). In addition, there were 34 red-fluorescent cells, which represented damaged or late apoptotic cells, as shown in Fig. 3d . To show the validity of the cytotoxicity assay result obtained by the partipetting-based method, we also measured the viability of the U2OS cells treated with drugs, using microtiter plate assays as reference data ( Fig. 3e ). The first reference was obtained by treating the cells with intact anticancer drugs as a control (blue bars in Fig. 3e ). We dispensed 100 μl of cells at 10 5 cells per ml into each well in a 96-well microtiter plate and incubated the cells for 24 h to allow cell attachment. The cells in each well were then treated with 100 μl of anticancer drug solution dissolved in serum-free culture medium. The concentrations of drugs used in the experiments in the microtiter plate were identical to the concentrations released from the ECMs, as listed in Table 1 . In addition, it was necessary to prove that the drugs released from the polymeric hydrogels were still effective against cancer cells because all of the drugs were first loaded into poly(ethylene glycol) diacrylate (PEG-DA) particles and then delivered to the cells by diffusion. Therefore, the second reference was obtained by the same method, but with treatment of the cells with drugs that were kept in contact with photopolymerized PEG-DA microparticles for 24 h (red bars in Fig. 3e ). As indicated by the green bars shown in Fig. 3e , the cell viabilities obtained by the partipetting-based assay were within ±17% of the results of the conventional method. Therefore, the results obtained using the partipetting-based multiplexed bioassay platform provide an acceptable range of cell viabilities compared with those acquired using a conventional assay approach. Scalable cell-based assay by partipetting The particle and cell chips used in the previous proof-of-concept experiments have ~400 microwells in a 30 × 30 mm chip ( Figs 2 and 3 ). We can apply the merits of the partipetting technique to perform a large-scale assay simply by increasing the size of the arrays. A multiplexed cytotoxicity assay was executed in a 76 × 52 mm chip with ~8,000 microwells to confirm the viability of the scaled-up partipetting scheme using four anticancer drugs: CPT, SS, PTX and PKF ( Fig. 4a ). 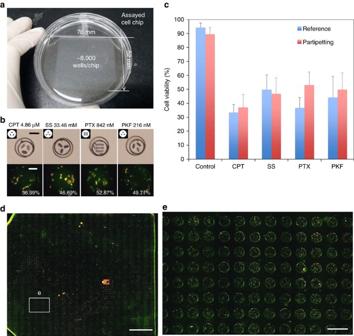Figure 4: A scalable multiplexed cytotoxicity assay by partipetting. (a) Photograph of the assayed cell chip. The size of both the particle and the cell chips was 76 × 52 mm, with ~8,000 microwells. (b) Four different drugs (CPT, SS, PTX and PKF) were loaded into microparticles and assembled in the microwells of a particle chip. The magnified view shows cells stained using an FITC Annexin V Apoptosis Detection Kit after 24 h of treatment with anticancer drug-loaded microparticles. Four different anticancer drugs, CPT, SS, PTX and PKF, were delivered to U2OS cancer cells using the scaled-up microwell platform. Scale bar, 100 μm. (c) Comparison between cell viabilities in conventional microtiter plates and in microwells treated using partipetting (n≥23; the error bars are means±s.d.) (d) Fluorescent microscopy image of the overall cell chip after staining using an apoptosis detection kit. Scale bar, 1 cm. (e) Magnified view of the assayed cells in each section. Scale bar, 1 mm. Figure 4b shows each ECM assembled in a microwell of the particle chip and the corresponding cell-based assay result in each case. The final concentrations of CPT, SS, PTX and PKF used to treat U2OS cells were 4.86 μM, 33.46 mM, 842 nM and 216 nM, respectively. The target cancer cells in the cell chip were reacted with the anticancer drugs released from each particle for 24 h and then stained using a FITC Annexin V Apoptosis Detection Kit to measure cell viability. We determined the cell viability of control and experimental groups treated with the same type and concentration of anticancer drug. Here, the control data, which represent a reference, were acquired using the conventional microtiter assay method, and the experimental data were obtained by the partipetting-based method. As observed in Fig. 4c , the results of the partipetting-based assay were within ±16% of the reference data. This finding implies that the partipetting-based assay provides results that are analogous to those obtained by a conventional method, even when the platform has been scaled up. Researchers in individual laboratories generally deliver each reagent to the assay platform by manually pipetting one at a time, but our assay method allows the delivery of 8,000 ECMs all at once, resulting in cost-effective and high-throughput bioassays. Figure 4: A scalable multiplexed cytotoxicity assay by partipetting. ( a ) Photograph of the assayed cell chip. The size of both the particle and the cell chips was 76 × 52 mm, with ~8,000 microwells. ( b ) Four different drugs (CPT, SS, PTX and PKF) were loaded into microparticles and assembled in the microwells of a particle chip. The magnified view shows cells stained using an FITC Annexin V Apoptosis Detection Kit after 24 h of treatment with anticancer drug-loaded microparticles. Four different anticancer drugs, CPT, SS, PTX and PKF, were delivered to U2OS cancer cells using the scaled-up microwell platform. Scale bar, 100 μm. ( c ) Comparison between cell viabilities in conventional microtiter plates and in microwells treated using partipetting ( n ≥23; the error bars are means±s.d.) ( d ) Fluorescent microscopy image of the overall cell chip after staining using an apoptosis detection kit. Scale bar, 1 cm. ( e ) Magnified view of the assayed cells in each section. Scale bar, 1 mm. Full size image Combinatorial cell-based assay by partipetting The partipetting-based bioassay technique is not confined to a one-to-one matching scheme, implying that a single cell well is aligned with a single particle well, as demonstrated in Figs 2 , 3 , 4 . More than one chemical can be delivered to the cells in each well simultaneously, thus enabling a combinatorial bioassay using the partipetting-based platform. Combinations of chemicals can be controlled according to the design of the placement of the microwell arrays in the particle chip. 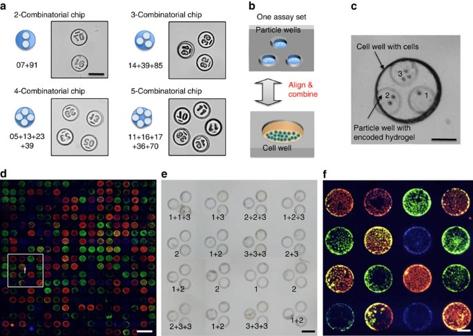Figure 5: Heterogeneous cell staining by combinatorial partipetting. (a) Various combinations of encoded microparticles in the particle chip. Microparticles with 100 different number codes were loaded and assembled in each particle chip, resulting in four different combinations of particles. Each combination of particles could be matched with a single microwell in the cell chip. Scale bar, 100 μm. (b) Schematic diagram of heterogeneous cell staining by three-chemical combinatorial partipetting. Three particle wells compose a single combination set in the particle chip, and this set is aligned and combined face-to-face with a single cell well of the cell chip, enabling various combinations of chemicals to be released in the target cell well. (c) Bright-field image of the combined particle and cell wells. Three different cell-staining dyes (orange, green and blue) are loaded into each encoded microparticle, and these ECMs are assembled in the particle chip for combinatorial partipetting. ‘1’, ‘2’ and ‘3’ represent the orange, green and blue CT-loaded microparticles, respectively. In one combination set, the cells in a single microwell are treated with three ECMs at the same time. (d) Fluorescence image of the assayed cell chip after the staining process by combining the particle and cell chips with the assembled CT-loaded microparticles (orange, green and blue CT dyes). Scale bar, 1 mm. (e,f) Matching of stained cells in the cell chip with each set of CT combinations in the particle chip. (e) Sectioned image from the particle chip. The numbers in the image represent each ECM fromFig. 5c. (f) Sectioned image from the cell chip in (d). The cells in each independent microwell of the cell chip were treated with three chemicals released from each combination set in the particle chip at the same time. Scale bars inFig. 5a–c,e,f, 200 μm. Figure 5a shows a particle chip whose combination consisted of 2, 3, 4 or 5 microwells in a circular formation. Microparticles with 100 different numerical codes were used to illustrate various potential combinations of chemicals. Thus, many different combinations of chemical substances can be used to perform assays together in a single microwell, as shown in Fig. 5a . Figure 5: Heterogeneous cell staining by combinatorial partipetting. ( a ) Various combinations of encoded microparticles in the particle chip. Microparticles with 100 different number codes were loaded and assembled in each particle chip, resulting in four different combinations of particles. Each combination of particles could be matched with a single microwell in the cell chip. Scale bar, 100 μm. ( b ) Schematic diagram of heterogeneous cell staining by three-chemical combinatorial partipetting. Three particle wells compose a single combination set in the particle chip, and this set is aligned and combined face-to-face with a single cell well of the cell chip, enabling various combinations of chemicals to be released in the target cell well. ( c ) Bright-field image of the combined particle and cell wells. Three different cell-staining dyes (orange, green and blue) are loaded into each encoded microparticle, and these ECMs are assembled in the particle chip for combinatorial partipetting. ‘1’, ‘2’ and ‘3’ represent the orange, green and blue CT-loaded microparticles, respectively. In one combination set, the cells in a single microwell are treated with three ECMs at the same time. ( d ) Fluorescence image of the assayed cell chip after the staining process by combining the particle and cell chips with the assembled CT-loaded microparticles (orange, green and blue CT dyes). Scale bar, 1 mm. ( e , f ) Matching of stained cells in the cell chip with each set of CT combinations in the particle chip. ( e ) Sectioned image from the particle chip. The numbers in the image represent each ECM from Fig. 5c . ( f ) Sectioned image from the cell chip in ( d ). The cells in each independent microwell of the cell chip were treated with three chemicals released from each combination set in the particle chip at the same time. Scale bars in Fig. 5 a – c , e , f , 200 μm. Full size image We demonstrated heterogeneous cell staining to show the potential of combinatorial bioassays using the partipetting-based platform. Each independent combination set was aligned and combined face-to-face with a single cell well in the cell chip, enabling combinatorial delivery of chemical substances to the target cells. Here each combination set consisted of three particle wells in a triangular formation, and this set was matched with one cell well ( Fig. 5b ). For ECMs, we loaded three different cell-staining dyes (orange, green and blue CT) into encoded hydrogels to visualize combinations of various dyes. The labels ‘1’, ‘2’ and ‘3’ in Fig. 5c represent orange, green and blue CT-loaded microparticles, respectively. Thus, when two chips were combined, the cells in a single microwell were simultaneously treated with three types of CT-loaded microparticles. Consequently, the cells could be stained with a combination of orange, green and blue dyes, including duplicated color combinations. Figure 5d shows the cell chip assayed with the particle chip, composed of randomly assembled orange, green and blue CT-loaded microparticles for combinatorial heterogeneous cell-staining experiments. The cells in each independent microwell were stained with a matching combination set, consisting of three CT-loaded microparticles. If two or three different CT dyes stained the same cells in the microwell, the fluorescence would merge the colors orange, green and blue, resulting in a color such as yellow, magenta, cyan or white. Figure 5e,f shows paired sets of particle and cell chips, with combinatorial heterogeneous cell staining. As shown in the representative fluorescence images in Fig. 5f , the mixed fluorescence of the cells indicates that the cells were successfully stained by a combination of CT-loaded microparticles from the set shown in Fig. 5e . In addition to combinatorial heterogeneous cell staining, we conducted a cytotoxicity assay using a three-chemical combinatorial particle chip. As shown in Fig. 6a , microparticles loaded with two different anticancer drugs were used, and each combination consisted of three particle wells in the particle chip, including microwells with no ECMs. This format allowed 10 different combinations of anticancer drugs in the particle chip (see concentrations in Table 2 ). Note that case 1 was classified as a control group because no ECMs were assembled in the combination set. 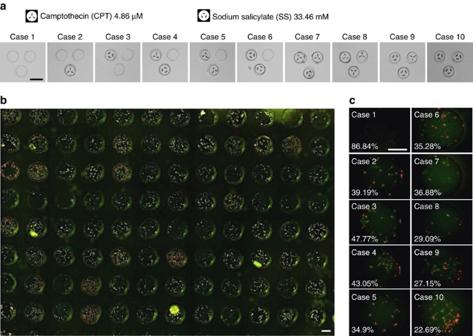Figure 6: A cytotoxicity test using a three-drug combinatorial particle chip. (a) Combination cases using two different anticancer drugs: camptothecin (CPT) and sodium salicylate (SS). A total 10 different combinations occurred in the particle chip, including microwells with no ECMs. Case 1 was a control group. (b) Fluorescence image of cells stained using an FITC Annexin V Apoptosis Detection Kit 24 h after combinatorial drug treatment in a three-drug combinatorial particle chip. (c) Each single cell well in the 10 combination cases. The mean measured value of cell viability in each case is denoted in the fluorescence images. Scale bars, 200 μm. Figure 6b,c shows a representative fluorescent image of cells stained using an FITC Annexin V Apoptosis Detection Kit after 24 h of treatment with combinatorial anticancer drugs. Here green and red fluorescence represents apoptotic and necrotic cells, respectively ( Supplementary Figs 8 and 9 ). Figure 6: A cytotoxicity test using a three-drug combinatorial particle chip. ( a ) Combination cases using two different anticancer drugs: camptothecin (CPT) and sodium salicylate (SS). A total 10 different combinations occurred in the particle chip, including microwells with no ECMs. Case 1 was a control group. ( b ) Fluorescence image of cells stained using an FITC Annexin V Apoptosis Detection Kit 24 h after combinatorial drug treatment in a three-drug combinatorial particle chip. ( c ) Each single cell well in the 10 combination cases. The mean measured value of cell viability in each case is denoted in the fluorescence images. Scale bars, 200 μm. Full size image Table 2 Concentrations of combinatorial anticancer drugs. Full size table To analyse cell viability in each drug-combination case, we needed to identify an address for each combination case in the particle chip and the target cells treated with the corresponding drug combination. For code mapping and data analysis, we developed an image-processing program using Python. We prepared overall images of a particle chip with randomly assembled ECMs and of an assayed cell chip, and the program then produced a map of codes for ECMs from the particle chip, a map of counted cells from the cell chip, and paired data from the particle chip and cell chip with calculated cell viabilities, as shown in Fig. 7a–d . We adopted the CellC algorithm to count viable and dead cells in fluorescent images [27] . The image processing required only a few minutes per chip, from decoding the assembled ECMs in the particle chip to mapping the cell viability data with the decoded drug-combination set. 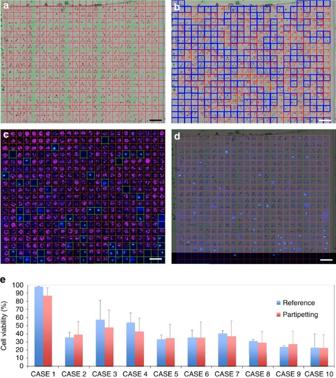Figure 7: Cell viability calculation from three-drug combinatorial partipetting data. (a) Particle chip with assembled ECMs for the combinatorial cytoxicity assay. Bright-field images ( × 4 microscope objective view) were arranged and stitched to obtain an overall particle chip image. The chip image was segmented into each combination by image processing. Microwells with ECMs were identified in this step. Each red circle represents a microwell with a particle. (b) Classification of combination cases and case counting. Each combination is classified by case, from 1 to 10. The red numbers are identified cases of each combination. The blue squares represent the cases that were filtered out as unrecognizable. Cases overlaid with both blue and red squares are modified cases that were initially identified incorrectly. (c) Cell chip segmented into individual microwells. To calculate the viabilities of cells treated with combinations of ECMs, cells were counted by image processing. The pink dots are cells recognized in each microwell. The green squares are segments that were filtered to remove errors. (d) Overlaid images of the particle and cell chips. Each combination case of the particle chip was paired with the corresponding microwells of the cell chip image. Scale bars, 1 mm. (e) Comparison of cell viabilities between conventional microtiter plates using pipetting and a microwell platform using partipetting. The blue bars in the graph represent the viabilities of cells reacted with drugs in microtiter plates as a reference. The red bars represent cell viabilities measured in the three-drug combinatorial partipetting platform. The data are within a maximum of ±10% of the conventional data (n≥43; the values are means+s.d.) Figure 7: Cell viability calculation from three-drug combinatorial partipetting data. ( a ) Particle chip with assembled ECMs for the combinatorial cytoxicity assay. Bright-field images ( × 4 microscope objective view) were arranged and stitched to obtain an overall particle chip image. The chip image was segmented into each combination by image processing. Microwells with ECMs were identified in this step. Each red circle represents a microwell with a particle. ( b ) Classification of combination cases and case counting. Each combination is classified by case, from 1 to 10. The red numbers are identified cases of each combination. The blue squares represent the cases that were filtered out as unrecognizable. Cases overlaid with both blue and red squares are modified cases that were initially identified incorrectly. ( c ) Cell chip segmented into individual microwells. To calculate the viabilities of cells treated with combinations of ECMs, cells were counted by image processing. The pink dots are cells recognized in each microwell. The green squares are segments that were filtered to remove errors. ( d ) Overlaid images of the particle and cell chips. Each combination case of the particle chip was paired with the corresponding microwells of the cell chip image. Scale bars, 1 mm. ( e ) Comparison of cell viabilities between conventional microtiter plates using pipetting and a microwell platform using partipetting. The blue bars in the graph represent the viabilities of cells reacted with drugs in microtiter plates as a reference. The red bars represent cell viabilities measured in the three-drug combinatorial partipetting platform. The data are within a maximum of ±10% of the conventional data ( n ≥43; the values are means+s.d.) Full size image Figure 7a,b shows the decoding process of the drug combinations in the particle chip. We first obtained bright-field images of the particle chip using a × 4 microscope objective view prior to the drug release step. In each × 4 image of the particle chip, we had a maximum of 20 combinations of particle wells, as indicated by the green rectangles. All green rectangles were arranged and stitched to a single chip image by image processing to obtain an overall particle chip image. Each microwell with an ECM was denoted as a red circle, and the total particle chip image was then segmented into individual combinations composed of three microwells by red grids ( Fig. 7a ). After the recognition of microwells filled with ECMs, each combination set was decoded and classified by its respective case, which is defined in Fig. 6a . Figure 7b shows all of the classified combination cases, from case 1 to case 10, in a single particle chip. Here the red numbers represent the identified combination cases, and the blue squares indicate cases classified as unrecognizable. The classified cases of drug combinations could be modified when the drug combinations were identified incorrectly, and these cases are overlaid with both red and blue squares. Similar to the particle chip segmentation, the cell chip image was also segmented into individual microwells by red grids to separately analyse cell viability in each microwell, as shown in Fig. 7c . The blue fluorescence indicates the total number of target cells, including both viable and dead cells that were stained with Hoechst 33342. A single cell chip had three independent images, blue, green and red fluorescence images, corresponding to total cells, apoptotic cells and necrotic cells, respectively, as previously explained in Fig. 3b . After segmentation of the cell chip into individual microwells, cells were recognized as pink dots and counted via image processing. Here the green squares are segments that were filtered to remove errors. Note that all of the blue, green and red fluorescence images were segmented by the same grid and counted to calculate cell viabilities according to each effective microwell ( Supplementary Fig. 8 ). Cell viability is defined as the percentage of living cells in each microwell. Finally, particle chip and cell chip images were matched to pair each combination case in the particle chip with the corresponding microwells of the cell chip ( Fig. 7d ). After eliminating unrecognizable particle codes in the particle chip and errors in the cell chip, all cell viabilities were matched with each drug-combination case in the particle chip. The viabilities of the cells assayed by the combinatorial partipetting approach were then compared with those of cells assayed by the conventional method to demonstrate the reliability of the combinatorial partipetting-based assay result ( Fig. 7e ). The blue bars in the graph represent the apoptotic viabilities of cells treated with drugs alone in microtiter plates as a reference. The red bars are apoptotic cell viabilities obtained using the three-drug combinatorial partipetting method. The results were within ±10% of those obtained by the conventional approach, showing the feasibility of a partipetting-based combinatorial cytotoxicity assay. In this study, we describe a partipetting-based bioassay platform using chemical-laden encoded microparticles. Partipetting potentially enables the handling of a large number of different chemicals in a single chip with a single operation and reagent cost reduction because of the sub-nanolitre volume of the hydrogel matrix. We demonstrated multiplexed and combinatorial cytotoxicity assays using cancer cell line and several anticancer drugs as simple applications of the partipetting-based approach. We believe that the partipetting technique is suitable for researchers who cannot afford an automated liquid handling system and huge reagent costs. Thus, compared with the manual pipetting method, our technique provides greater opportunities to perform large-scale quantitative assays in individual laboratories. Owing to its simplicity and flexibility, we envision that the proposed method will encourage innovation in the development of a wide range of various bioassays, including cell-based assays, enzymatic assays and protein–protein interaction studies, and a host of other future applications. ECM fabrication Encoded microparticles are fabricated in a high-throughput manner by an optofluidic maskless lithography (OFML) technique [29] , which enhances variations in graphical codes by dynamic masking via a digital micromirror device (DMD). The OFML system allows the encoding of hydrogels for drug identification by manipulating the DMD pattern during in situ photopolymerization ( Supplementary Fig. 1 ). The code for each particle, which is a mask of DMD, is designed individually using the program Paint (Microsoft Windows, USA) and uploaded to the DMD software of the OFML system. The hydrogels are selectively photopolymerized by exposure to UV radiation at 100% intensity with a 0.1 s curing time through the × 10 objective lens of the OFML system. Here each microparticle has a diameter of 180 μm and a thickness of 60 μm. All of the fabricated hydrogel particles are first collected in ethyl alcohol (EtOH) solution. To prevent the photoinitiator residue of uncured resin from inducing cell death inside the hydrogels, we repeat the washing with fresh EtOH solution to thoroughly wash the particles and then vortex mix or sonicate the hydrogels two to three times. We then let the particles sink to the bottom of the EtOH solution for a few minutes, after which we remove the EtOH. Next, the particles are placed in anti-adhesion dishes (that is, Falcon tube caps) or tubes. To completely remove any EtOH remaining around the microparticles, we dry them in a desiccator overnight or in an oven for 30 min at 50 °C. Materials We used poly(ethylene glycol) diacrylate (PEG-DA, M n =700; Sigma-Aldrich) with 5 wt% photoinitiator (2-hydroxy-2-methylpropiophenone 97%, Sigma-Aldrich) to synthesize the polymeric structures. To demonstrate heterogeneous cell staining, we loaded 0.2 mM CT Red CMPTX, Orange CMTMR, Green CMFDA or Blue CMF 2 HC (Invitrogen) into the encoded microparticles. In the multiplexed cytotoxicity assays, we used anticancer drugs, including camptothecin (CPT, M n =348.4; Sigma-Aldrich), sodium salicylate (SS, M n =160.11; Sigma-Aldrich), paclitaxel (PTX, M n =853.91; Sigma-Aldrich), auranofin (AF, M n =679.5; Sigma-Aldrich) and PKF118-310 (PKF, M n =193.16; Sigma-Aldrich). For mixed drug treatments, CPT and SS were blended at ratios of 1:1, 1:2 and 2:1 to illustrate drug repositioning [27] , [28] . The microparticles were stored and handled in mineral oil (Sigma-Aldrich) or silicone oil (Sigma-Aldrich) during the partipetting process. Measurement of released anticancer drug concentration We prepared the set of 100,000 ECMs for each type of anticancer drug in duplicate. We used five anticancer drugs for the concentration measurements: CPT (MW=348.4), SS (MW=160.11), PKF (MW=193.16), PTX (MW=853.91) and AF (MW=853.91). During the partipetting process, a single ECM is exposed to target cells in an individual cell well. The dimensions of a microwell in the cell chip are 500 μm (diameter) by 300 μm (depth), giving the microwell a volume capacity of 59 nl. Therefore, for each set of drugs, 100,000 microparticles are reacted with 5.9 ml of buffer (that is, DI water). After 24 h of drug release, we extracted the drug-containing buffer to measure the drug concentrations. For the reference calibration curve, we measured the light absorbance of several known concentrations of each drug. The reference drugs used for the concentration measurements were drug solutions that were kept in contact with photopolymerized PEG-DA microparticles. We measured the light absorbance of unknown drug concentrations and fit the values to a reference calibration curve. In this way, we determined the final concentrations of drugs released into the buffer solution. Supplementary Fig. 7 shows the light absorbance graphs of each drug in DI water, including the reference and test data. In each graph, all the unknown and known concentrations of drugs are plotted. We compared the absorbance peaks at specific wavelengths to determine the concentration of each drug released into the buffer. Drug release curve To estimate a predictable drug concentration when a drug diffuses into medium, we generated a drug-release reference curve based on actual concentrations of released drugs. Supplementary Fig. 7b shows an example: the drug-release reference curve of SS at 12 different drug-loading concentrations, which was used to assess the drug’s release tendency. We first fabricated SS-loaded microparticles at 12 drug-loading concentrations: 0.2, 1, 2, 10, 20, 50, 100, 200 and 500 mM, and 1, 2 and 3 M. Note that the solubility of SS in water is up to 660 g l −1 , yielding a drug concentration of 4.1 M. In addition, the PEG-DA microparticles in this experiment were fabricated using 100% UV intensity in the OFML system. Each concentration set has 15,000 microparticles, and these particles were reacted with 885 μl of DI water for 24 h. We then measured the light absorbance of DI water to determine the released drug concentration. The concentration of drug released from ECMs is controllable within the linear range from 0.2 mM to 1 M for the loading concentration of SS. The concentration of released drug then saturates at a loading concentration of ~1 M, a limit imposed by the maximum absorption capacity of the hydrogel matrix. Cell culture U2OS human osteosarcoma cells (KCLB, Korean Cell Line Bank) were cultured in McCoy’s 5A culture medium with 1% penicillin–streptomycin and 10% fetal bovine serum at 37 °C under 5% CO 2 and 95% atmospheric air. Cultured cells were detached from culture flasks by trypsinization using 0.25% trypsin and 0.13% EDTA in phosphate-buffered saline. The cells were centrifuged and dispersed in cell culture medium to produce a cell density of ~10 5 cells per ml. All of the PDMS microwell plates (both cell chips and particle chips) were first sterilized in an autoclave for 20 min at 120 °C, followed by oxygen plasma treatment for 1.5 min. The disinfected microwell plates were treated with fibronectin (Sigma-Aldrich) for 45 min to enhance cell adhesion on and protein absorption to the PDMS microwell plates. Release of chemicals and apoptosis assay A cell chip with attached target cells in the microwells was aligned and placed face-to-face with the corresponding particle chip containing partipetted ECMs using a microscope. The assembled chips were then fixed with paper clips and incubated for 24 h to allow sufficient drug release by diffusion and apoptosis induction by the anticancer drugs. After reaction with the drugs, the cell chip was gently washed five times with phosphate-buffered saline and stained with an apoptosis-detecting solution (FITC Annexin V Apoptosis Detection Kit, BD Pharmingen) and membrane-permeable DNA-staining dye (Hoechst 33342, Invitrogen) for 20 min in an incubator. How to cite this article: Chung, S. E. et al. One-step pipetting and assembly of encoded chemical-laden microparticles for high-throughput multiplexed bioassays. Nat. Commun. 5:3468 doi: 10.1038/ncomms4468 (2014).